Trapping atoms using nanoscale quantum vacuum forces Quantum vacuum forces dictate the interaction between individual atoms and dielectric surfaces at nanoscale distances. For example, their large strengths typically overwhelm externally applied forces, which makes it challenging to controllably interface cold atoms with nearby nanophotonic systems. Here we theoretically show that it is possible to tailor the vacuum forces themselves to provide strong trapping potentials. Our proposed trapping scheme takes advantage of the attractive ground-state potential and adiabatic dressing with an excited state whose potential is engineered to be resonantly enhanced and repulsive. This procedure yields a strong metastable trap, with the fraction of excited-state population scaling inversely with the quality factor of the resonance of the dielectric structure. We analyse realistic limitations to the trap lifetime and discuss possible applications that might emerge from the large trap depths and nanoscale confinement. One of the spectacular predictions of quantum electrodynamics is the emergence of forces that arise purely from quantum fluctuations of the electromagnetic vacuum [1] . Also known as London-van der Waals [2] or Casimir forces [3] in different regimes, these forces are often dominant at short distances and can give rise to undesirable effects in nanoscale systems, such as nanomechanical stiction [4] . These forces have also attracted increasing attention in the fields of atomic physics and quantum optics. In particular, significant efforts have been made in recent years to interface cold atoms with the evanescent fields of dielectric micro- and nano-photonic systems [5] , [6] , [7] , [8] , [9] , [10] , [11] , [12] , [13] , [14] . These systems are expected to facilitate strong, tunable interactions between individual atoms and photons for applications such as quantum information processing [15] and the investigation of quantum many-body physics [16] , [17] , [18] . In practice, efficient atomic coupling to the evanescent fields of the nanophotonic systems requires that atoms be trapped within sub-wavelength distances of these structures. At these scales, quantum vacuum forces can overwhelm the forces associated with conventional optical dipole traps, typically resulting in a loss of trap stability at distances d ≲ 100 nm from dielectric surfaces. Given the ability to engineer the properties of nanophotonic structures, an interesting question arises as to whether such systems could be used to significantly modify vacuum forces, perhaps changing their sign from being attractive to repulsive, or even creating local potential minima. The strength of nanoscale vacuum forces should lead to unprecedented energy and length scales for atomic traps, which would find use beyond nanophotonic interfaces, such as in quantum simulation protocols based on ultracold atoms [19] and control of inter-atomic interactions [20] . Here we propose a novel mechanism in which engineered vacuum forces can enable the formation of a nanoscale atomic trap. While a recent no-go theorem [21] forbids a vacuum trap for atoms in their electronic ground states, tailored nanophotonic systems can yield strong repulsive potentials for atomic excited states. We show that a weak external optical field can give rise to an overall trapping potential for a dressed state. Remarkably, absent fundamental limits on the losses of the surrounding dielectric structure, the fraction of excited-state population in the dressed state can become infinitesimal, which greatly enhances the trapping lifetime and stability. We identify and carefully analyse the actual limiting mechanisms. While we present calculations on a simple model where analytical results can be obtained, we also discuss the generality of our protocol to realistic systems such as photonic crystal structures. Quantum interactions between atom and surface The no-go theorem for non-magnetic media states that a dielectric object in vacuum cannot be stably trapped with vacuum forces for any surrounding configuration of dielectric objects, provided that the system is in thermal equilibrium [21] . In analogy with Earnshaw’s theorem, which prohibits trapping of charged objects with static electric potentials, at best one can create a saddle-point potential (see, for example, ref. 22 involving metal particles and refs 13 , 23 for a hybrid vacuum/optical trap for atoms). For dielectric objects, potential loopholes involve embedding the system in a high-index fluid [24] or using blackbody radiation pressure associated with strong temperature gradients [25] . Applied to atoms, this theorem essentially forbids the stable vacuum trapping near a dielectric structure when the atom is in its electronic ground state. No such constraint exists for atoms in their excited states [26] , although the robustness of any possible trap would be limited by the excited-state lifetime. Here, we show that an atom only weakly dressed by its excited state can be trapped by properly tailoring the dispersion of the underlying structure. We begin by briefly reviewing how quantum vacuum fluctuations give rise to forces on the ground and excited states. Within an effective two-level approximation of an isotropic atom with ground and excited states | g ›, | e ›, respectively, the interaction between the electromagnetic field and an atom at position r is given by the dipole Hamiltonian H =− d · E ( r ). Conceptually, following a complete decomposition of the electric field into its normal modes k , one can write , where . The energy non-conserving terms ( and ) enable an atom in its ground state | g , 0› to couple virtually to the excited state and create a photon, | e , 1 k ›, which is subsequently re-absorbed. The corresponding frequency shift for the ground state within second-order perturbation theory is δω g ( r )=−∑ k g k ( r ) 2 /( ω 0 + ω k ), where ω 0 is the unperturbed atomic transition frequency. This shift results in a vacuum-induced mechanical potential when translational symmetry is broken owing to dielectric surfaces. Using a quantization technique for electrodynamics in the presence of dispersive dielectric media, the shift can be expressed in terms of the scattered component of the dyadic electromagnetic Green’s function evaluated at imaginary frequencies ω = iu (ref. 27 ) (also see Methods), where Γ 0 is the free-space spontaneous emission rate of the atom. For simplicity, we have given the result in the zero-temperature limit. Finite-temperature corrections [28] , [29] associated with atomic interactions with thermal photons are only relevant for distances from surfaces comparable with or larger than the thermal blackbody wavelength, d ≳ λ T , where at T =300 K. A similar process can occur for an atom in its excited state | e , 0›, in which the atom virtually emits and re-absorbs an off-resonant photon (thus coupling to the state | g , 1 k ›). However, the excited state is unique in that it can also emit a resonant photon. The total excited-state shift is given by [27] The first term arises from off-resonant processes, while the second term can be interpreted as the interaction between the atom and its own resonantly emitted photon. Naturally, the dielectric environment can modify the spontaneous emission rate as well, Note that the resonant shifts and modified emission rates are complementary, in that they emerge from the real and imaginary parts of the Green’s function. Micro- and nano-photonic systems are already widely exploited to modify emission rates of atoms and molecules in a variety of contexts [30] , [31] , [32] , [33] . We propose that these same systems can be used to tailor excited-state potentials to facilitate vacuum trapping. Interactions with a Drude material In what follows, we present a simple model system that enables one-dimensional trapping in a plane parallel to a semi-infinite dielectric slab, as illustrated in Fig. 1 . The use of a homogeneous dielectric (as opposed to, for example, a photonic crystal) greatly simplifies the calculation and enables one to understand the relevant trap properties analytically, although we later argue why the qualitative features should still hold in more complex, realistic settings. In the dielectric slab model, dispersion engineering will be realized via the frequency-dependent electric permittivity ε ( ω ). While this particular system achieves a one-dimensional trap along z , our electrodynamic calculations are performed in three dimensions. 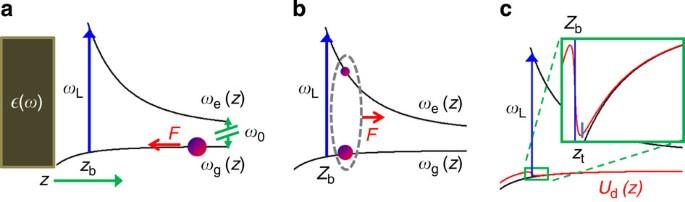Figure 1: Schematic of vacuum trapping mechanism. (a) A semi-infinite dielectric with specially tailored frequency-dependent permittivity ε(ω) enables large repulsion in the excited stateωe(z), in contrast to the attractive vacuum potential experienced by an atom in its ground state. An overall trapping potential normal to the surface (alongz) can be generated by driving the atom with an external laser of frequencyωL, which is greater than the natural resonance frequencyω0of the atom. The laser comes into local resonance with the atom atzb. An atom far fromzbis unaffected owing to the large laser detuningωL−ω0and feels an attractive forceFtoward the dielectric interface. (b) The atom comes closer to local resonance with the laser asz→zb. This creates an atomic-dressed state, whose excited-state component yields a net repulsive force on the atom. (c) A slowly moving atom experiences the adiabatic dressed-state potentialUd(z) shown in red, which characterizes the position-dependent mixing between ground and excited states. The minimum of the dressed potential is located atzt>zb. Figure 1: Schematic of vacuum trapping mechanism. ( a ) A semi-infinite dielectric with specially tailored frequency-dependent permittivity ε( ω ) enables large repulsion in the excited state ω e ( z ), in contrast to the attractive vacuum potential experienced by an atom in its ground state. An overall trapping potential normal to the surface (along z ) can be generated by driving the atom with an external laser of frequency ω L , which is greater than the natural resonance frequency ω 0 of the atom. The laser comes into local resonance with the atom at z b . An atom far from z b is unaffected owing to the large laser detuning ω L − ω 0 and feels an attractive force F toward the dielectric interface. ( b ) The atom comes closer to local resonance with the laser as z → z b . This creates an atomic-dressed state, whose excited-state component yields a net repulsive force on the atom. ( c ) A slowly moving atom experiences the adiabatic dressed-state potential U d ( z ) shown in red, which characterizes the position-dependent mixing between ground and excited states. The minimum of the dressed potential is located at z t > z b . Full size image A short-distance expansion of the Green’s function, valid for sub-wavelength scales, shows that the excited-state emission rate Γ( z ) and resonant contribution to the shift are given by where the permittivity ε a = ε ( ω 0 ) is evaluated at the atomic resonance frequency, z is the distance from the surface and k 0 = ω 0 / c is the resonant free-space wavevector. A large repulsive potential is generated when ε a approaches −1 from above, ε a →−1 + , which is analogous to the interaction between a classical dipole at position z and its large induced image dipole in the dielectric. The modified spontaneous emission rate originates from the absorption or quenching of the atomic emission owing to material losses. We choose a Drude model, , as a simple dielectric function. Note that this function satisfies Kramers–Kronig relations (causality), as a choice of a non-causal function could result in an apparent violation of the no-go theorem [21] as well. In the limit of vanishing material loss parameter γ , the system passes through ε =−1 at the plasmon resonance frequency . The system is conveniently parameterized by the quality factor Q ≡ ω pl / γ and a dimensionless detuning Δ p =( ω − ω pl )/ γ . For Q >>Δ p , the factor resembles the complex susceptibility of a simple resonator, which in the far-detuned limit (Δ p >>1) yields and . The dispersion and dissipation scale like and , respectively. Thus, for high Q , it is possible to choose detunings where the atom still sees significant repulsive forces, but where spontaneous emission into the material is not significantly enhanced (in addition to material-induced emission of equation (4), there still is emission into free-space at a rate ∼ Γ 0 ). This scaling behaviour is in close analogy with conventional optical trapping of atoms, where simultaneously using large trapping intensity and detuning maintains reasonable trap depths but suppresses unwanted photon scattering. The ground-state shift for atomic frequencies ω 0 ∼ ω pl and in the near-field is given by . An additional condition for the validity of the short-distance results obtained for the excited state is , as shown in the Methods. We continue to present approximate results in this regime owing to its simplicity, although all of our numerical results (such as in Figs 2c,d and 3 ) are calculated using the full Green’s functions. 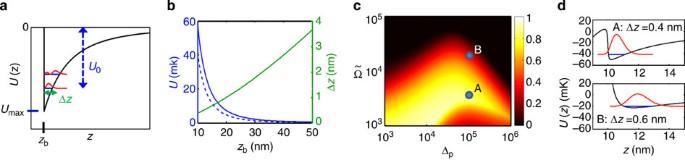Figure 2: Trap properties. (a) Ideal limit of trapping potential, corresponding to the pure ground-state potentialħδωg(z) and an infinite barrier atz=zb. The maximum depth of the potential is denoted byUmax≡ħ|δωg(zb)|. The quantum wavefunction amplitudes |ψ(z)|2(in arbitrary units) for the two lowest eigenstates are illustrated in red, while the binding energyU0and position uncertainty Δzof the ground state are depicted as well. (b) Properties of the ideal trapping potential versus barrier positionzb, for the case of a Caesium atom. The blue solid and dashed curves give the potential depth at the barrier position,Umax, and the ground-state-binding energyU0, respectively. The green curve depicts the ground-state uncertainty Δz. (c) For the non-ideal trapping potential, the depth of the classical potentialUdepthis numerically calculated. Here we plot it normalized by the maximum possible valueUmax≡ħ|δωg(zb)|, versus detuning parameter Δpand normalized Rabi freuqency. (d) The trapping potential, ground-state-binding energyU0, and wavefunction amplitude |ψ(z)|2for the parameter sets A, B, as illustrated inc. The colour coding is the same as ina. Figure 2: Trap properties. ( a ) Ideal limit of trapping potential, corresponding to the pure ground-state potential ħδω g ( z ) and an infinite barrier at z = z b . The maximum depth of the potential is denoted by U max ≡ ħ | δω g ( z b )|. The quantum wavefunction amplitudes | ψ ( z )| 2 (in arbitrary units) for the two lowest eigenstates are illustrated in red, while the binding energy U 0 and position uncertainty Δ z of the ground state are depicted as well. ( b ) Properties of the ideal trapping potential versus barrier position z b , for the case of a Caesium atom. The blue solid and dashed curves give the potential depth at the barrier position, U max , and the ground-state-binding energy U 0 , respectively. The green curve depicts the ground-state uncertainty Δ z . ( c ) For the non-ideal trapping potential, the depth of the classical potential U depth is numerically calculated. Here we plot it normalized by the maximum possible value U max ≡ ħ | δω g ( z b )|, versus detuning parameter Δ p and normalized Rabi freuqency . ( d ) The trapping potential, ground-state-binding energy U 0 , and wavefunction amplitude | ψ ( z )| 2 for the parameter sets A, B, as illustrated in c . The colour coding is the same as in a . 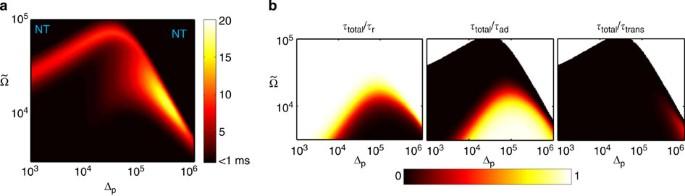Figure 3: Trap lifetime. (a) Trap lifetimeτtotalversus dimensionless Rabi frequencyand detuning Δp. Here we have assumed a plasmon resonance quality factor ofQ=107and atomic properties corresponding to Caesium. The regions of parameter space where no trap exists are labelled ‘NT’ in the plot. (b) For the same parameters, the individual contributions of recoil heating, anti-damping and transient heating are plotted as a fraction of the total heating rate. Tunnelling contributes less than 10−2to the total heating over this range of parameters and is not plotted here. Full size image Figure 3: Trap lifetime. ( a ) Trap lifetime τ total versus dimensionless Rabi frequency and detuning Δ p . Here we have assumed a plasmon resonance quality factor of Q =10 7 and atomic properties corresponding to Caesium. The regions of parameter space where no trap exists are labelled ‘NT’ in the plot. ( b ) For the same parameters, the individual contributions of recoil heating, anti-damping and transient heating are plotted as a fraction of the total heating rate. Tunnelling contributes less than 10 −2 to the total heating over this range of parameters and is not plotted here. Full size image We also briefly comment on two effects in realistic systems that can be safely excluded from our analysis. First, in principle, the excited-state shift can be affected by coupling to even higher electronic levels. However, a careful calculation of this contribution [34] shows that it is negligible compared with the resonantly enhanced term of equation (5), provided that we work in the regime Q >>Δ p . Second, we have ignored corrections to the shifts owing to surface roughness. It can be shown that the length scale for modifications to the shifts is roughly set by the size of the surface variation itself [35] . The realistic regimes of operation of our trap will be at d ≳ 10 nm from surfaces, which allows us to safely ignore the angstrom-scale surface roughness achievable in state-of-the-art dielectric structures [36] . Formation of a vacuum trap We now describe how a trap can form for an atom subject to these potentials, and in the presence of a weak driving laser of frequency ω L and Rabi frequency Ω (see Fig. 1 ). For conceptual simplicity, we choose the Rabi frequency to be spatially uniform, such that all atomic forces are attributable to the vacuum potentials alone. Qualitatively, the strong position dependence of the ground- and excited-state frequencies causes the laser to come into resonance with the atom at a single, tunable point z = z b . Under certain conditions (described in detail later), an atom starting at position z >> z b will be far detuned, such that it is essentially in the ground state and is attracted by the pure ground-state potential. However, moving closer to z b brings the atom closer to resonance. The dressing of the atom with a small fraction of excited-state population causes a repulsive barrier to form near z ∼ z b , yielding a metastable trap. Significantly, our approach does not attempt to directly counteract the attractive ground-state potential with large external optical potentials, in sharp contrast with other trapping schemes near dielectric surfaces [8] , [9] , [11] , [12] , [37] , [38] , [39] . The order of our calculation of the trap properties is as follows. We first find the adiabatic potential experienced by a slowly moving atom. We derive relevant properties around the location of the trap minimum z t ( Fig. 1 ). In particular, we show that absent material constraints (arbitrarily high Q ), the dressed state can in principle have infinitesimal excited-state population and scattering. We then quantize the motion to find the motional eigenstates, binding energy and position uncertainty Δ z . Finally, we analyse the mechanisms that limit the trap lifetime. Following standard procedures [40] , the average force experienced by the atom is given by the expectation value of the Heisenberg equation , while the internal atomic dynamics satisfies the usual Bloch equations, for example, Here, for notational simplicity, denotes the expectation value of the atomic variables, and we have defined δ a ( z )= ω L −( ω e ( z )− ω g ( z )) as the detuning between the laser and the local atomic resonance frequency. When the atom moves slowly on the timescales of the internal dynamics, the atomic coherence can be adiabatically eliminated, , such that the atomic populations are functions of position alone, . We are primarily interested in the regime where the atom is weakly driven, σ ee <<1. A more careful calculation reveals that the Green’s function G sc ( r , r , ω ) for the excited-state resonant shift and emission rate in equations (2) and (3) must in fact be evaluated at the laser frequency in this regime, which reflects that the atom primarily acts as a Rayleigh scatterer (see Methods). Consequently, ε a in equations (4) and (5) is replaced with ε ( ω L ). The adiabatic potential seen by a slowly moving atom is . In principle, the Heisenberg equation for should also include the effects of spontaneous emission. It can be shown, however, that this term contributes a zero average force (see Methods), and only results in a heating term to be analysed later. Three independent frequencies characterize the system ( ω L , ω p and ω 0 ), and two relative frequencies must be specified. One is determined by selecting the trap barrier position, determined by the relation δ a ( z b )≡0. A second is the dimensionless detuning between the plasmon resonance and laser, Δ p =( ω L − ω pl )/ γ , which we treat as a free parameter that determines the relative strengths of the excited-state shift and dissipation. In the near-field, the excited-state repulsion exceeds the ground-state attraction by a factor 2 Q /3Δ p . The population at z b must then exceed the inverse of this quantity, σ ee >3Δ p /2 Q , to provide a classical barrier in the adiabatic potential, which translates to a minimum Rabi frequency . Since Δ p ≲ Q , this scheme potentially enables atom trapping near surfaces with greatly reduced intensities as compared with conventional trapping. In the latter case, an optical dipole potential requires a minimum driving field of to overcome the attractive ground-state potential. The excited-state population at the trap minimum is fixed by the ratio of ground to excited-state forces, , and is surprisingly independent of Ω (provided that Ω>Ω min ). An increasing Rabi frequency has the effect of increasing the local detuning δ a ( z t ) to preserve the same population. This manifests itself as a self-selection of the trapping position and an increasing distance from the barrier with increasing intensity, where we have defined the dimensionless Rabi frequency . The ability to tune the trap position using both the laser amplitude and its frequency (which determines z b ) enables the adiabatic transformation between deep but small traps close to the surface to larger, shallow traps ∼ 100 nm from the surface. This is expected to greatly facilitate trap loading, as techniques to trap atoms at these larger distances are already well established [8] , [11] , [12] , [41] . The photon-scattering rate at the trap position, R sc =Γ( z t ) σ ee ( z t ), leads to lifetime limitations of our trapping scheme. Fixing other parameters, the detuning Δ p from the plasmon resonance can be optimized to yield the minimum scattering rate, . Thus, absent fundamental limits on the magnitude of Q , the photon-scattering rate can in principle be suppressed to an arbitrary degree. This implies that an infinitesimal violation of the assumptions underlying the no-go theorem can in fact allow for trapping. In a conventional optical dipole trap, the potential U =− α ( ω L )| E ( r , ω L )| 2 /2 seen by an atom depends on the local field intensity and is proportional to a spatially constant atomic polarizability evaluated at the laser frequency. In contrast, here we exploit a novel mechanism arising from strong spatial variations in the polarizability itself, induced through the vacuum level shifts. This creates a back-action effect analogous to that producing a dynamical ‘optical spring’ in opto-mechanical systems [42] , and enables extremely steep trap barriers around z b (as in Fig. 1c ). In particular, the repulsive force is given by , where is engineered to be large. However, the excited-state population itself varies strongly with position through the spatially dependent detuning (for simplicity, here we omit the varying linewidth Γ( z )). Taking into account the spatial variation of σ ee around the equilibrium position, one finds an overall repulsive force that scales like , Results for trapping of caesium Given the possible steepness of this barrier, an ideal limit for the overall potential is shown in Fig. 2a . The attractive part consists of the pure ground-state potential and arises from quantum fluctuations, while an infinite hard wall is created at z = z b owing to the combination of strong resonant excited-state shifts (originating from the interaction of the atom with a classical image dipole) and opto-mechanical back-action. This idealized model enables one to understand the best possible scaling of the trap properties. In particular, the trap depth U depth (the energy required for a classical particle to become unbound) cannot exceed the value of the ground-state potential at z b , U max ≡ ħ | δω g ( z b )| (for example, U max ≈60 mK when z b =10 nm for a Caesium atom). This trapping potential can be easily quantized numerically. In Fig. 2b , we plot the quantum-binding energy U 0 (where 0< U 0 < U depth ≤ U max ) and position uncertainty Δ z for the motional ground-state wavefunction. For the numerical results in Figs 2 and 3 , we use atomic properties corresponding to Caesium ( λ 0 =852 nm, Γ 0 /2 π =5.2 MHz, recoil frequency ω r /Γ 0 =4 × 10 −4 ). The strength of the vacuum potentials is reflected in the strong confinement of the wavefunctions (for example, Δ z <4 nm for distances z b <50 nm), which are an order of magnitude smaller than in conventional optical traps. To contrast our results for Caesium with those of a less massive atom, we have considered Lithium as well. Results for Li similar to those for Cs in Fig. 2a,b show that at z b =10 nm, the potential depth is smaller by roughly a factor of two, while the confinement Δ z sees roughly a fivefold increase. Generally, within the Wentzel–Kramers–Brillouin approximation and to lowest order in Δ z , the ground-state localization scales like k 0 Δ z ∼ ( ω r ( k 0 z b ) 4 /Γ 0 ) 1/3 , while the binding energy U 0 ≈ U max (1−3Δ z/z b ) can be nearly the entire classical potential depth. This ideal model describes qualitatively well the actual potentials over a large parameter regime. In Fig. 2c , we plot the ratio of the numerically obtained trap depth to the theoretical maximum, U depth / U max , as functions of Δ p and dimensionless driving amplitude . Here, we have chosen a quality factor of Q =10 7 and a barrier position of z b =10 nm. A trap depth comparable with U max is achievable over a large range of values. For low values of , the trap depth is weakened owing to escape over the potential barrier, while for large values, the trap becomes shallow as its position z t is pulled away from z b (as discussed previously). Two representative trap potentials, along with the ground-state wavefunctions and confinement Δ z are illustrated in Fig. 2d . Analysis of trap heating We have identified four sources of motional heating—recoil heating, non-adiabatic motion of the atom within the trap, fluctuations of the atomic coherence and tunnelling over the finite-height potential barrier—that limit the trap lifetime in absence of external cooling mechanisms. Tunnelling is exponentially suppressed with barrier height and thus is easily suppressed with increasing Rabi frequency. This calculation can be found in the Methods, while we discuss the more important mechanisms here. As in conventional optical trapping, the random momentum recoil imparted on the atom by scattered photons yields an increase in motional energy at the rate . Two qualitative differences emerge relative to free space, however. First, the photon-scattering rate is modified in the presence of dielectric surfaces. Second, the effective momentum ħk eff imparted by a photon is enhanced compared with the free-space momentum. This momentum scales at close distances like (see Methods), owing to emission of high-wavevector photons into the dielectric. Starting from the motional ground state, this heating causes the atom to become unbound over a timescale τ r ≈( k 0 z t ) 2 Δ p /(3 ω r ). It should be noted that the heating rate d E /d t does not depend on the atom confinement (that is, whether we operate in the Lamb-Dicke limit), as the suppression of motional jumps in tight traps is compensated by the increase in energy gained per jump [43] . The increase in lifetime with trap position, , is attributable entirely to the reduction in recoil energy associated with a photon emitted into the surface. In particular, the decreasing trap depth versus distance is exactly compensated for by the reduced surface-enhanced emission rate . Our derivation of the atomic potential assumes that the atomic coherence adjusts rapidly to the local trap properties, d σ ge /d t ≈0, which results in a purely conservative potential. As we now show, non-adiabatic corrections result in a momentum-dependent force, d p /d t ∝ p (anti-damping). We can solve equation (6) for the atomic motion perturbatively by writing , where is the adiabatic solution. It depends only on the instantaneous position and is given by in the weak saturation limit. Here, δ c ( z )= δ a ( z )+ i Γ( z )/2 is the complex detuning. Substituting this solution into equation (6) yields a velocity-dependent correction to the coherence, . This in turn yields a new contribution to the force, F (1) = βp , where the anti-damping rate is given by evaluated at the trap position z t . Intuitively, the atom is anti-damped ( β >0) because the laser frequency is blue-detuned relative to the atomic frequency at z t , giving rise to preferential Stokes scattering over anti-Stokes. Aside from the term proportional to dΓ/d z , the heating rate is exactly analogous to that occurring in an opto-mechanical system in the blue-detuned regime [42] . We define a characteristic time τ ad needed for the energy increase produced by anti-damping to equal the ground-state-binding energy U 0 . Thus far, we have focused on the motion of the atomic-dressed state, in which a trap emerges owing to weak mixing with the excited-state potential. Following a spontaneous emission event, however, the atom returns to the ground state and sees the pure ground-state potential for a transient time t trans ∼ | δ c ( z t )| −1 until the atomic coherence is restored, during which the atomic wave packet accelerates toward the surface and gains energy. While a simulation of the full dynamics of the atom (including the spatial and internal degrees of freedom) is quite challenging, here we estimate the heating rate from these transient processes. In particular, we first find the spatial propagator under the pure ground-state potential, U ( z f , z i , t f , t i ) (see Methods). Then, assuming that a spontaneous emission event occurs at t i =0 with the atom initially in the motional ground state ψ ( z i ), the new wavefunction that emerges once the coherence equilibrates is given by ψ ( z f ) ∼ ∫d z i U ( z f , z i , t trans , 0) ψ ( z i ). The probability of atom loss P trans per spontaneous emission event is estimated from the overlap between the initial and final states, P trans =1−|‹ z f | z i ›| 2 , with a corresponding trap lifetime of . The overall trap lifetime is obtained by adding the individual lifetimes in parallel, , and is plotted in Fig. 2a . The overall trap lifetime exhibits a complicated dependence on Rabi frequency Ω and detuning Δ p owing to the different scalings of the constituent heating mechanisms (see Fig. 3b ). As an example, however, for external parameters Δ p =2.5 × 10 5 and Ω/Ω min =1.5 × 10 4 for atomic Cs, one achieves a lifetime of τ total ≈15 ms, ground-state confinement of Δ z ≈1 nm, trap depth of U depth ≈10 mK and trap distance of z t ≈15 nm. This Rabi frequency corresponds to an incident intensity of just 0.05 mW μm −2 . To compare, nanofibre-based optical traps [8] , [11] employ guided intensities three orders of magnitude larger to achieve confinement and surface distances of Δ z ∼ 20 nm (corresponding to trap frequencies of ) and z t ∼ 200 nm, respectively. Trapping frequencies of ω m /2 π ≈40 MHz would be needed to reach single-nanometer confinement, far beyond what is realistic in optical traps. An additional heating mechanism, which does not appear in our simple model of an isotropic two-level atom, arises from the possibility of an excited state in a realistic multi-level atom to emit photons of different polarizations and transition into different states in a ground-state manifold. The different Clebsch–Gordan coefficients of these transitions, along with the symmetry breaking introduced by the nearby dielectric structure, imply that different excited states can experience different vacuum shifts. This would appear as different trapping potentials for the various dressed ground-state sub-levels absent of some special engineering. As a result, spontaneous changes in the sub-levels (such as arising from spontaneous photon scattering) would induce fluctuations of the trapping potential and lead to motional heating. One possibility to prevent these issues in an experiment is to utilize the effective two-level structure provided by a cycling transition. We have described a protocol for an atomic trap based on engineered vacuum forces, and have analysed in detail a model case of one-dimensional trapping near a Drude material, where analytical results are possible to obtain. The Drude response approximates well a number of metals, such as silver and gold, in the optical domain [44] . In practice, however, these metals are limited by their low-quality factors ( Q <10 2 ), and the thermal fluctuations of such conducting materials can give rise to strong noise-induced trap heating and decoherence [45] . On the other hand, photonic crystal structures enable engineering of resonances through geometry, and quality factors approaching Q ∼ 10 7 have been observed [46] . We anticipate that our trapping protocol could be quite generally applied, and the resulting trap behaviour would qualitatively remain the same. In particular, the spatial dependence of the excited-state properties would no longer scale like ( k 0 z ) −3 as in the case of a simple dielectric surface, but be characterized by a more complex spatial function f ( r ) that reflects the mode shape of the underlying structure [23] . However, the scaling of the excited-state shift ( δω e ∝ Q /Δ p ) and emission ( ) is generic to coupling between an atom and resonator of Lorentzian lineshape, and thus the capability of achieving highly stable traps with high- Q structures using our proposed techniques is maintained. Photonic crystals thus offer great flexibility in tailoring the properties of vacuum traps (such as dimensionality), which we plan to investigate in detail in future work. For example, it has been shown that dielectric gratings can produce quantum vacuum forces that trap atoms along the lateral directions of a dielectric interface [35] , which when combined with our previous techniques could yield full three-dimensional traps. We note that theoretical [23] and experimental efforts [13] have already been made to achieve realistic hybrid atom traps in photonic crystal structures, where a combination of vacuum forces and optical forces is required to stabilize the trap in all dimensions. In addition, while we have focused on trapping of atoms weakly dressed by an external laser, it would be interesting to investigate the feasibility of laser-free traps, where atoms pumped into metastable electronic levels are stably confined using engineered resonant shifts alone. The ability to create atomic traps with parameter sets (such as depth, confinement and proximity to surfaces) that are not possible in conventional traps (whether optical, electrical or magnetic) should lead to a number of intriguing applications. For example, it has been proposed that the trapping of atoms near dielectric surfaces with nanoscale features (such as a sub-wavelength lattice) would facilitate large interaction strengths and long-range interactions for ultracold atoms [39] . However, the major limitation of optical trapping is the divergent intensity needed to overcome the ground-state vacuum forces of these structures. The use of resonantly enhanced excited-state repulsion to create a trap could significantly reduce the power requirements and enable smaller lattice constants. Furthermore, traps with localization on the nanometer scale can induce inter-atomic forces that are of comparable strength with molecular van der Waals forces, which enables novel opportunities to control ultracold atomic collisions [20] and realize exotic interactions such as p -wave scattering of fermions [47] . Atoms trapped near surfaces could also act as exquisite nanoscale probes of surface physics, including the precision measurement of vacuum forces themselves. Electromagnetic field quantization In this section, we briefly describe the quantization scheme of the electromagnetic field in the presence of arbitrary linear dielectric media, which follows that of ref. 27 . The free field is characterized by a set of bosonic modes with frequencies ω and annihilation operators ( j = x , y , z ), with a corresponding Hamiltonian The bosonic operators satisfy canonical commutation relations and are physically associated with noise polarization sources in the material. The electric field operator at frequency ω is driven by the sources at the same frequency and is given in the Coulomb gauge by [27] Here and in the following, it is assumed that all repeated vector or tensor indices are summed over, for example, is the frequency-dependent permittivity at position r , and G ij is the dyadic Green’s function which is the (gauge-invariant) solution to The total electric field is E ( r )=∫d ω E ( r , ω )+h.c. Similarly, the magnetic field is . It can be verified that these expressions preserve the same field commutation relations as in free-space field quantization. We now consider a two-level atom at position r a and with ground and excited states | g ›, | e ›, respectively, interacting with the electromagnetic field within the electric dipole approximation. The interaction Hamiltonian is given by where is the atomic dipole matrix element. Plane-wave expansion We consider an interface with vacuum in the region z >0 and a dielectric with permittivity ε ( ω ) in the region z <0. The solution to equation (11) in the region z >0 can be written as the sum of a free component (that is, the solution in isotropic vacuum) and a scattered component. In the region 0≤ z ≤ z ′, they can be expanded in plane waves, which yields Here k || =( k x , k y ) and ρ =( x , y ) are the wavevector and position along the direction parallel to the interface, while the full wavevector is given by with the relation . Further defining as the perpendicular component of the wavevector in the medium, and are the Fresnel reflection coefficients for s and p polarized waves, respectively. Ground-state interactions The interaction Hamiltonian H af couples the ground state of the bare system | g , 0› (consisting of the atomic ground state and vacuum) to states . Within second-order perturbation theory, this interaction induces a shift of the bare ground-state energy by an amount where ω 0 is the bare resonance frequency of the atom. Substituting equations (10) and (13) into the expression above, and using analyticity of the integrand to rotate the frequency integral onto the positive imaginary axis ω = iu , one finds [27] Here, we have only included the scattered component of the Green’s function, as the free component gives a contribution that is independent of position. While we have considered a two-level atom for simplicity, a more realistic model of an isotropic atom consists of multiple excited states and equal polarizabilities in each direction (that is, the ground state can emit virtual photons of any polarization with equal strength). Since the contribution to the ground-state shift from each excited-state transition is additive, equation (17) can be modified to account for this by setting for all i and associating with the free-space spontaneous emission rate of any excited state. This yields equation (1). Excited-state interactions We want to analyse the effective excited-state properties in the specific case that an atom is weakly driven by a classical field of frequency ω L . We thus transform to a rotating frame where the free atomic evolution is given by and δ = ω L − ω 0 is the detuning between the laser frequency and atomic resonance frequency ω 0 . The standard technique to derive the excited-state shift and decay rate follows that of the ground state and uses time-independent second-order perturbation theory [27] . In this approach, however, one cannot find the jump operator associated with photon emission, which is needed to calculate the effect of emission on atomic motion (for example, recoil heating). To rectify this, we employ an alternative approach based on deriving an atomic master equation within the Born–Markov approximation [48] . In particular, the equation of motion for the reduced atomic density matrix ρ a is given by where is the interaction Hamiltonian in the interaction picture (with respect to the free Hamiltonian H 0 = H a + H f ) and |0› is the electromagnetic vacuum state. Any exponential of time appearing in the integral can be evaluated using the relation . Using the field expansion of equation (10) in and following some manipulation, equation (18) can be written in the form The effective Hamiltonian describes coherent interactions between the atom and vacuum field and takes the form which can be interpreted as a position-dependent energy shift of the excited state. Taking a simple isotropic two-level model for an atom, the excited-state shift is found to be as stated in the main text. The Liouvillian term [ ρ a ] can be written in a Lindblad form The jump operators take the form The excited-state spontaneous emission rate is in turn given through the relation , or This again averages over dipole orientations and reproduces equation (3), with the replacement of ω 0 → ω L . To derive this, we have used the identity The expressions for the excited-state emission rate Γ( r a ) and level shift δω e ( r a ) agree with previous derivations [27] , if the laser frequency ω L is replaced by the atomic resonance frequency ω 0 . The appearance of ω L physically describes the effect of the weakly driven atom (that is, a linear optical element) interacting with its own Rayleigh-scattered field, which can be altered owing to the presence of nearby dielectric surfaces. This is in accordance with the well-known result for the fluorescence spectrum of a driven atom, which is dominated by the Rayleigh contribution for atomic populations σ ee <<1 (ref. 48 ). More importantly, we have obtained for the first time a decomposition of the jump operator associated with photon emission for arbitrary dielectric surroundings, which enables one to calculate recoil heating. Short-distance limit We now derive the short-distance expansion of the excited-state properties. The resonant term in equations (2) and (3) depend on the quantity Tr G sc ( r a , r a , ω L ), which for planar interfaces is given by For short distances, the expression is dominated by large k || ≈ ik ⊥ , which gives rise to a long exponential tail . Expanding to second order for large k || , this tail contributes as We now apply these results to the Drude model. First, we note the exact relation . For frequencies within a range Δ p ≲ Q of the plasmon resonance, one readily finds that the response is well approximated by a complex Lorentzian. For larger detunings Δ p ≳ Q , the exact expression of ε ( ω ) must be used. Furthermore, within the range Δ p ≲ Q , one must compare the size of the first and second terms on the right-hand side of equation (27). The first term dominates the integral provided that , in which case which reproduces the asymptotic expressions for the excited-state shift and linewidth in the main text. Tunnelling The atomic escape rate from the metastable potential formed by the vacuum trapping scheme owing to quantum tunnelling is calculated in the Wentzel–Kramers–Brillouin approximation in two steps. First, we find an approximation to the real part of the bound-state energy ħω b . This is implemented by replacing the actual metastable-dressed-state potential U d ( z ) with a stable one, U s ( z ), according to the formula (also see Fig. 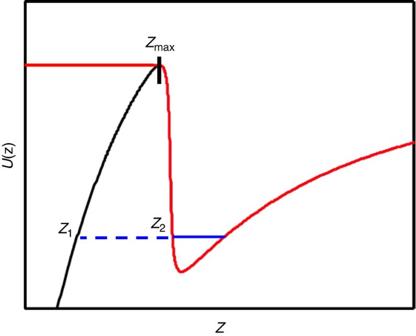Figure 4: Tunnelling. Black curve: metastable-dressed-state potentialUd(z) (in arbitrary units) seen by the atom. The maximum of the metastable barrier is located atzmax. Red curve: stable potentialUs(z) used to approximately calculate the binding energyħωb(blue line) of the atom in the trap. The classical turning pointsz1, 2of a particle with this energy, which are used to evaluate the tunnelling rate in the Wentzel–Kramers–Brillouin approximation, are labelled as well. 4 ) Figure 4: Tunnelling. Black curve: metastable-dressed-state potential U d ( z ) (in arbitrary units) seen by the atom. The maximum of the metastable barrier is located at z max . Red curve: stable potential U s ( z ) used to approximately calculate the binding energy ħω b (blue line) of the atom in the trap. The classical turning points z 1, 2 of a particle with this energy, which are used to evaluate the tunnelling rate in the Wentzel–Kramers–Brillouin approximation, are labelled as well. Full size image Here, z max is the position corresponding to the maximum of the metastable barrier. The ground-state energy of U s ( z ) is solved numerically. Once the approximate ground-state-binding energy is obtained, the tunnelling probability P t for a particle hitting the metastable barrier is calculated using the Wentzel–Kramers–Brillouin approximation, Here, z 1,2 are the solutions to U d ( z )= ħω b and are thus the classical turning points of a particle with energy ħω b . The rate that the trapped atom collides with the barrier is approximated by Δ p z / m Δ z , where the position and momentum uncertainties are obtained from the numerical ground-state solution. We then estimate the inverse of the tunnelling-limited lifetime to be . Recoil heating Recoil heating can be calculated by treating the atomic position r a in equation (23) as an operator. For notational simplicity, we shall consider recoil heating only along the trapping direction z , although our results can be easily generalized. The increase in momentum uncertainty owing to photon scattering is given by Here we will focus solely on the Liouvillian term in the density matrix evolution (that is, momentum incurred from spontaneous emission). It can be shown that the Liouvillian term produces no net force, that is, . Using the fact that for any function f , one can derive the following general expression for the recoil heating rate in terms of Green’s functions, Here, the derivatives ∂ 1 and ∂ 2 act on the first and second spatial arguments of the Green’s functions, respectively, and we have suppressed the atomic spatial variables in the directions that are not of interest. We further assume that the internal and spatial degrees of freedom can be de-correlated, . This is valid in our regime of interest where properties such as the excited-state decay rate have negligible variation over the spatial extent of the atomic wave packets. As in the main text, we use the notation to denote the expectation value of atomic operators. Formally, we can write the above equation in the convenient form This form is intuitive as it describes the momentum increase arising from a random walk process, where the atom experiences random momentum kicks of size ± ħk eff at a rate Γ( r a ) σ ee (that is, the photon-scattering rate). k eff is a derived quantity that thus characterizes the effective momentum associated with scattered photons in the vicinity of a dielectric surface. As a simple example, we consider an atom in free space polarized along x . Evaluating equation (33) with the free-space Green’s function G free,xx from equation (14) yields (and Γ( r a )=Γ 0 ), recovering the known result [43] . This recoil momentum is smaller than the full momentum ω L / c of the scattered photon because the atom emits in a dipole pattern, but only the projection of the photon momentum along z contributes to motional heating in that direction. Applying the same formalism to an atom near a dielectric described by the Drude model, we find that the scattered component of the Green’s function dominates the recoil heating, leading to the asymptotic expansion of given in the main text. In all of our numerical calculations, the full Green’s function is used rather than asymptotic results. Transient heating Following a spontaneous emission event, the spatial wavefunction of the atom is temporarily untrapped and evolves under the pure ground-state potential for a characteristic time t trans before the internal dynamics equilibrates. Here we derive an approximate propagator U ( z f , z i , t f , t i ) for the wavefunction evolving under the ground-state potential. The problem significantly simplifies if the ground-state potential U g ( z )= ħω g ( z ) is linearized around the atom trapping position z = z t , This linearization is justified in our regime of interest where the atom is tightly trapped and the wavefunction undergoes little evolution in the time t trans . The constant energy and position offsets in the Hamiltonian play no role, and thus we can consider the simplified Hamiltonian . The propagator for this Hamiltonian is given by where is the well-known propagator for a free particle [49] . In our simulations, the ground-state wavefunction for an arbitrary trapping potential is obtained numerically on a lattice, and so the propagator must be spatially discretized as well. In particular, while the exponential term in equation (36) is well-behaved on a lattice, the free propagation U free is not at short times. We instead replace U free with the propagator D mn ( t ) for the free discrete Schrodinger equation, where β = ħ /2 ma 2 , n is the lattice site index, and a is the lattice constant. The propagator for this equation (defined as the matrix satisfying ψ m ( t )= D mn ψ n (0)) is given by where J n is the n -th order Bessel function. How to cite this article: Chang, D. E. et al. Trapping atoms using nanoscale quantum vacuum forces. Nat. Commun. 5:4343 doi: 10.1038/ncomms5343 (2014).